Use of trifluoroacetaldehyde N-tfsylhydrazone as a trifluorodiazoethane surrogate and its synthetic applications Trifluorodiazoethane (CF 3 CHN 2 ), a highly reactive fluoroalkylating reagent, offers a useful means to introduce trifluoromethyl groups into organic molecules. At present, CF 3 CHN 2 can only be generated by oxidation of trifluoroethylamine hydrochloride under acidic conditions; due to its toxic and explosive nature, its safe generation and use remains a prominent concern, hampering wider synthetic exploitation. Here we report the development of trifluoroacetaldehyde N-tfsylhydrazone (TFHZ-Tfs) as a CF 3 CHN 2 surrogate, which is capable of generating CF 3 CHN 2 in situ under basic conditions. The reaction conditions employed in this chemistry enabled a difluoroalkenylation of X–H bonds (X = N, O, S, Se), affording a wide range of heteroatom-substituted gem -difluoroalkenes, along with Doyle-Kirmse rearrangements and trifluoromethylcyclopropanation reactions, with superior outcomes to approaches using pre-formed CF 3 CHN 2 . Given the importance of generally applicable fluorination methodologies, the use of TFHZ-Tfs thus creates opportunities across organic and medicinal chemistry, by enabling the wider exploration of the reactivity of trifluorodiazoethane. Trifluorodiazoethane (CF 3 CHN 2 , also known as trifluoromethyldiazomethane) is a highly reactive trifluoromethylating agent employed in transformations such as cycloadditions [1] , [2] , [3] , [4] , [5] , [6] , X–H insertions [7] , [8] , coupling reactions [9] , [10] and homologations (Fig. 1 a) [11] , [12] . CF 3 CHN 2 is generated by the oxidation of trifluoroethylamine hydrochloride (CF 3 CH 2 NH 2 ·HCl) under acidic conditions, but being a toxic and explosive gas, handling of CF 3 CHN 2 at room temperature is extremely hazardous if a significant buildup occurs [2] , [13] . Although first described in 1943 [14] , only in the last decade have improvements to this method been made, involving slow addition of aqueous NaNO 2 to trifluoroethylamine to avoid an accumulation of large amounts of CF 3 CHN 2 [2] . More recently, other operational improvements have been developed, such as the small-scale preparation of CF 3 CHN 2 in solution [5] , [7] , [8] , the recycling of gaseous CF 3 CHN 2 [9] , and the use of continuous-flow chemistry [15] , [16] , [17] . Nevertheless, the use of specifically designed equipment and/or operating conditions remains a general limitation, and reagents that are easily handled but capable of slowly generating CF 3 CHN 2 in situ under mild conditions (ideally complementing current oxidative/acidic methods) are of high appeal. Fig. 1 Generation and transformations of trifluorodiazoethane, and synthesis of TFHZ-Tfs. a Synthesis and applications of trifluoromethyldiazomethane (CF 3 CHN 2 ) in organic synthesis. CF 3 CHN 2 is a highly reactive trifluoroalkylation reagent, but its simplex synthesis method, inherent toxicity and explosiveness limit its widespread application. Because of its hazardous nature, manifold methods have been developed for the safer use of CF 3 CHN 2 such as slow addition of oxidants, small-scale preparation of CF 3 CHN 2 solution, recycling of gaseous CF 3 CHN 2 and continuous-flow chemistry. b Method for the generation of CF 3 CHN 2 from trifluoroacetaldehyde N-tfsylhydrazone under basic condition and gem -difluoroalkenylation of X–H Full size image We targeted the use of trifluorinated N-sulfonylhydrazones as a trifluorodiazoethane surrogate. As a class of stable precursors to diazo compounds, sulfonylhydrazones are widely used in synthesis [18] , [19] , [20] , [21] , [22] ; however, trifluoroacetaldehyde-derived sulfonylhydrazones have not been explored as surrogates for CF 3 CHN 2 [23] , [24] . gem -Difluoroalkenes are important motifs in the design of mechanism-based enzyme inhibitors, and as bioisosteres of the carbonyl group [25] , [26] , [27] , and are typically prepared by Wittig or Julia–Kocienski-type reactions [28] , [29] , [30] , or by cross-coupling [31] , [32] , [33] , [34] . However, these methods are mostly effective only for the synthesis of C -substituted gem -difluoroalkenes, while the synthesis of their heteroatom-substituted counterparts is comparatively rare and suffers from narrow substrate scope, or requires strong bases or toxic reagents [35] , [36] , [37] , [38] , [39] . We report here the development of trifluoroacetaldehyde N-tfsylhydrazone (TFHZ-Tfs) as a bench-stable CF 3 CHN 2 precursor, which decomposes in a controlled manner under basic conditions to release CF 3 CHN 2 into the reaction system (Fig. 1b ); this strategy circumvents the need for slow addition or manual handling of CF 3 CHN 2 , thus minimizing exposure and reducing the potential explosion risk. Importantly, this base-mediated approach also led to the discovery of novel reactivity of CF 3 CHN 2 : we describe its use in the difluoroalkenylation of X–H (X = N, O, S, Se) bonds, overcoming limitations in previous routes to these motifs, and also in Doyle–Kirmse and cyclopropanation reactions, which display excellent stereoselectivity and yields, and collectively demonstrate the potential utility of TFHZ-Tfs as a trifluorodiazoethane surrogate. Synthesis of TFHZ-Tfs TFHZ-Tfs could be easily accessed by condensation of the o -trifluoromethylbenzenesulfonyl hydrazide with trifluoroacetaldehyde monohydrate under acidic conditions. The reaction proved readily scalable, TFHZ-Tfs could be prepared in high yield (91%) on 85 mmol scale as a bench-stable crystalline solid, and in a cost-effective manner, which is attractive for synthetic applications. In addition, TFHZ-Tfs could be stored at ambient temperature for at least 5 months without degradation (as characterized by 1 H NMR spectroscopy). Investigation of reaction conditions An exploration of the reactivity of TFHZ-Tfs began in the difluoroalkenylation of X–H bonds. p -Methylthiophenol was identified as a suitable nucleophile for this study, and to our delight we found that in the presence of aqueous KOH, sodium dodecylbenzenesulfonate (SDBS, 30 mol%), and the iron porphyrin catalyst FeTPPCl (5 mol%) in dichloromethane at 40 °C, TFHZ-Tfs delivered the difluoroalkenylated product 2 in 51% yield, along with 9% of the trifluoroethyl thioether 2′ (Fig. 2 , Entry 1). Iron porphyrin complexes have been applied as highly efficient catalyst in carbene-transfer reactions [40] . Screening of other iron porphyrin complexes led to the discovery of the more robust Fe[P2] catalyst, which at just 1 mol% loading afforded 2 in 80% isolated yield, while suppressing the formation of side product 2′ (Entries 2 and 3). Under the same conditions, TFHZ-Ns and TFHZ-Ts gave 2 in significantly lower yield (Entries 4 and 5). Additional optimization of this S–H gem -difluoroalkenylation led to refinement of the reactions parameters (Entry 3, TFHZ-Tfs (2.0 equiv), 5 mL KOH aq. 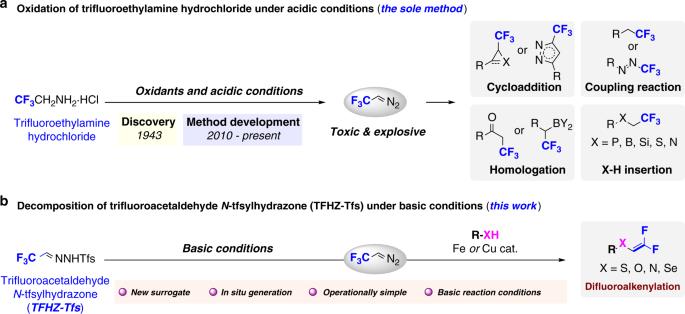Fig. 1 Generation and transformations of trifluorodiazoethane, and synthesis of TFHZ-Tfs.aSynthesis and applications of trifluoromethyldiazomethane (CF3CHN2) in organic synthesis. CF3CHN2is a highly reactive trifluoroalkylation reagent, but its simplex synthesis method, inherent toxicity and explosiveness limit its widespread application. Because of its hazardous nature, manifold methods have been developed for the safer use of CF3CHN2such as slow addition of oxidants, small-scale preparation of CF3CHN2solution, recycling of gaseous CF3CHN2and continuous-flow chemistry.bMethod for the generation of CF3CHN2from trifluoroacetaldehyde N-tfsylhydrazone under basic condition andgem-difluoroalkenylation of X–H (20 wt%), and SDBS (30 mol%) in the presence of 1 mol% of Fe[P2] in DCM at 40 °C under air; see Supplementary Table 1 for details). Fig. 2 Optimization of the iron-catalyzed gem -difluoroalkenylation of p -methylthiophenol with trifluoromethyl sulfonylhydrazones. Reaction conditions: thiophenol (0.3 mmol), sulfonylhydrazone (0.6 mmol), Fe porphyrin catalyst, SDBS (sodium dodecylbenzenesulfonate) (0.09 mmol), DCM (1.0 mL), and KOH solution (5.0 mL, 20% wt %), 40 °C, 18 h, under air. a Yields determined by 1 H NMR spectroscopic analysis with CH 2 Br 2 as an internal standard. b Reaction carried out under Ar atmosphere. c Yield in parentheses is the isolated yield Full size image Scope of thiol gem- difluoroalkenylation Having established the decomposition profile of TFHZ-Tfs, and conditions for thiol difluoroalkenylation, the scope of this insertion was explored. Under the optimized conditions of Fig. 2 Entry 3 (Method A), a broad tolerance of arene substituents was observed (Fig. 3 ), with thiophenols bearing both electron-donating and electron-withdrawing substituents giving the corresponding difluoroalkenes in good to excellent yields ( 2 – 19 ). Notably, reaction efficiency was not compromised by the positioning of the aryl substituent ( ortho , meta , or para ), and indeed sterically hindered mono- or bis- ortho- substituted substrates afforded the difluoroalkenes in high yields ( 20 – 21 ). Thienyl, furyl, and 2-naphthalene thiols were also excellent substrates, leading to heteroaryl- and naphthyl sulfides 22 – 24 . We were pleased to find that benzeneselenol performed equally well, affording the selenodifluoroalkene 25 in 66% yield. The difluoroalkenylated structure was unambiguously confirmed by single crystal X-ray diffraction analysis of sulfone 9′ , which was prepared by oxidation of 9 with m -CPBA (see Supplementary Table 7 for X-ray crystallographic data). Fig. 3 Scope of gem -difluoroalkenylation of X–H (X = N, O, S, Se). 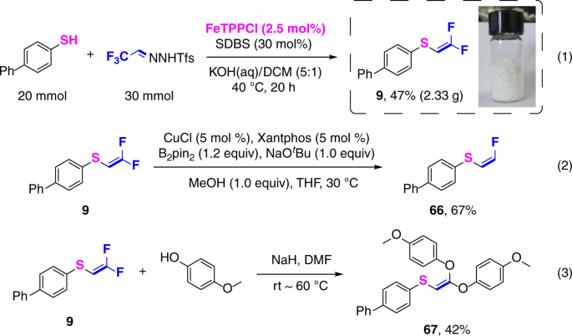Fig. 4 Gram-scale synthesis and further transformations. Gram-scale synthesis of product9(1). Mono-defluorination of product9(2). Double defluorination of product9(3) 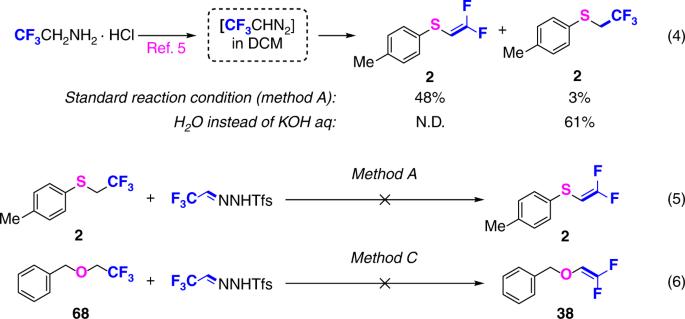Fig. 5 Mechanistic investigations. Base promotes fluoride elimination (4) Intermediate experience verification (5) and (6) 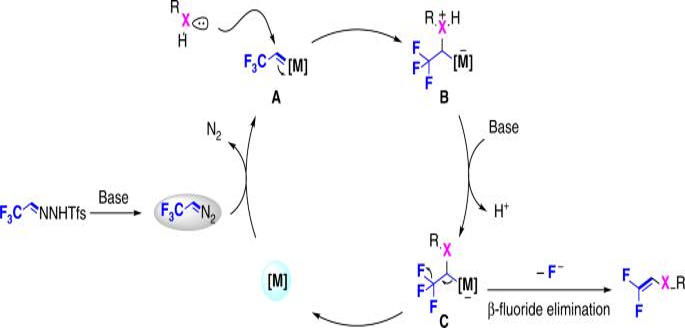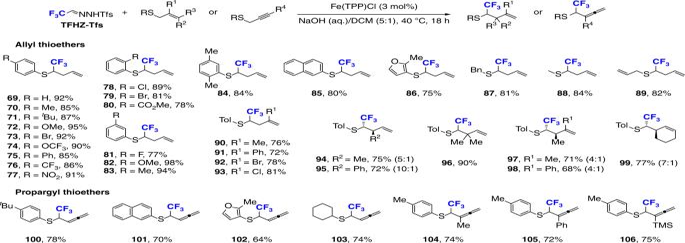Fig. 7 Scope of Doyle–Kirmse reaction. Reaction conditions: thioether (0.3 mmol), TFHZ-Tfs (0.6 mmol), FeTPPCl (3 mol%), NaOH (aq.)/DCM (5:1), 40 °C, 18 h Fig. 6 Proposed mechanism. Mechanistic insights regarding to formation of oxonium ylide and fluoride elimination 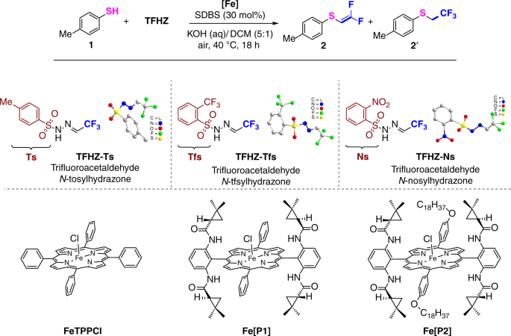Reaction conditions: Method A: thiophenol (0.3 mmol), TFHZ-Tfs (0.6 mmol), Fe[P2] (1 mol%), SDBS (30 mol%), KOH (aq. )/DCM (5:1), air, 40 °C, 18 h. Method B: amine (0.3 mmol), TFHZ-Tfs (0.6 mmol), Cu(OTf) 2 (20 mol%), LiO t Bu (4 equiv), DCE: toluene (3:1), Ar, 40 °C, 24 h. Method C: TFHZ-Tfs (1.0 mmol), NaH (4 equiv) and DCE (8.0 mL) were stirred at rt for 1 h under Ar, then CuBr (30 mol%), alcohol (0.5 mmol), and LiO t Bu (1 equiv) were added and the mixture was stirred at 40 °C under Ar for 24 h. *Reaction performed for 30 h. † Number in parentheses is the yield based on recovered starting material (brsm). ‡ The yield was determined by 1 H NMR spectroscopic analysis with CH 2 Br 2 as an internal standard Full size image Scope of amine gem- difluoroalkenylation We next questioned whether other heteroatoms could also serve as suitable nucleophilic coupling partners, and turned our attention to amine difluoroalkenylation. After extensive screening of reaction parameters, a copper catalyst system was identified that efficiently mediated this transformation, consisting of Cu(OTf) 2 (20 mol%) and LiO t- Bu (4.0 equiv) in DCE:toluene (3:1) under argon at 40 °C (Fig. Fig. 2 Optimization of the iron-catalyzedgem-difluoroalkenylation ofp-methylthiophenol with trifluoromethyl sulfonylhydrazones. Reaction conditions: thiophenol (0.3 mmol), sulfonylhydrazone (0.6 mmol), Fe porphyrin catalyst, SDBS (sodium dodecylbenzenesulfonate) (0.09 mmol), DCM (1.0 mL), and KOH solution (5.0 mL, 20% wt %), 40 °C, 18 h, under air.aYields determined by1H NMR spectroscopic analysis with CH2Br2as an internal standard.bReaction carried out under Ar atmosphere.cYield in parentheses is the isolated yield 3 , Method B, see Supplementary Table 2 for details of reaction optimization). The reaction scope encompassed a variety of aniline derivatives, with ring substituents including halides, nitriles, ketones, esters, and anthraquinones, delivering the gem -difluoroenamines in moderate to good yields ( 26 – 35 ). 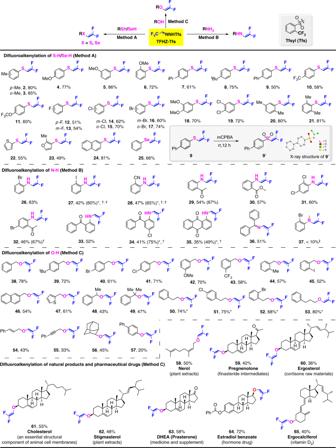In some cases, incomplete conversions were observed, but the residual amine substrate could be recovered. In addition to primary anilines, benzophenone imine proved a viable substrate: product 36 was obtained in 51% yield, suggesting this method could be applied to the N-difluoroalkenylation of other nitrogen-based nucleophiles. Secondary amines did not prove suitable, as shown by the low yield of compound 37 . Scope of alcohol gem- difluoroalkenylation Further expansion of the scope of the methodology was achieved through modification of the copper catalyst to enable the synthesis of difluorovinyl ethers from alcohols (Fig. Fig. 3 Scope ofgem-difluoroalkenylation of X–H (X = N, O, S, Se). Reaction conditions: Method A: thiophenol (0.3 mmol), TFHZ-Tfs (0.6 mmol), Fe[P2] (1 mol%), SDBS (30 mol%), KOH (aq.)/DCM (5:1), air, 40 °C, 18 h. Method B: amine (0.3 mmol), TFHZ-Tfs (0.6 mmol), Cu(OTf)2(20 mol%), LiOtBu (4 equiv), DCE: toluene (3:1), Ar, 40 °C, 24 h. Method C: TFHZ-Tfs (1.0 mmol), NaH (4 equiv) and DCE (8.0 mL) were stirred at rt for 1 h under Ar, then CuBr (30 mol%), alcohol (0.5 mmol), and LiOtBu (1 equiv) were added and the mixture was stirred at 40 °C under Ar for 24 h. *Reaction performed for 30 h.†Number in parentheses is the yield based on recovered starting material (brsm).‡The yield was determined by1H NMR spectroscopic analysis with CH2Br2as an internal standard 3 , Method C, for details of optimization see Supplementary Table 3 ). A wide selection of benzyl-, alkyl-, and heteroaryl-substituted alcohols afforded gem -difluorovinyl ethers in good to excellent yields; for benzyl alcohols, the position of substituents on the arene had little influence on the reaction outcome ( 38 – 47 ), and secondary and tertiary benzyl alcohols also afforded the corresponding products with respectable efficiency ( 48 and 49 ). Alkyl alcohols (such as phenethyl and phenylpropyl), and other functionalized alcohols (such as cinnamyl, propargyl, and 2-adamantyl), all proved reactive partners, affording products 50 – 56 in moderate to high yields. In contrast to aliphatic alcohols, phenols showed poor reactivity; for example, 4-biphenylol gave the difluoroalkenylated product 57 in just 20% yield, which presumably reflects the poorer nucleophilicity of the phenol compared to the aliphatic substrate. Scope of gem- difluoroalkenylation with bioactive molecules To illustrate potential utility, the methodology was applied to the gem -difluoroalkenylation of selected natural products, drugs, and pharmaceutical intermediates. For instance, various terpene and steroid natural products (nerol, pregnenolone, ergosterol, cholesterol, and stigmasterol) were derivatized into the desired difluorovinyl ethers in good yields ( 58 – 63 ). Estradiol benzoate, a highly potent hormone therapy agent used to treat estrogen deficiencies, could also be converted to the corresponding gem -difluoroalkenylated product 64 in 72% yield. Further, the synthesis of gem -difluoroalkenylated vitamin D 2 65 , (the parent being a potent drug for treatment of cutaneous tuberculosis and lupus erythematosus), was achieved in the presence of its potentially sensitive triene functionality, underlining the functional group tolerance of this methodology. It is notable that fluoroalkyl ethers represent the key structure of many insecticides and lubricants; the ready availability of such gem -difluorovinyl ethers may provide new opportunities for the design and construction of such molecules [41] . Gram-scale synthesis and further transformations For multigram-scale applications, the Fe[P2] catalyst (which requires a multistep synthesis) could be conveniently replaced with the commercially available FeTPPC1 (Fig. 4 ). Using this alternative catalyst with dichloromethane as solvent, gem -difluorovinyl sulfide 9 was obtained in a yield of 47%, which is comparable to that obtained with Fe[P2] (Method A, 50%). Interestingly, this product could be smoothly mono-defluorinated by treatment with CuCl and B 2 pin 2 to give the ( Z )-monofluorovinyl sulfide 66 in 67% yield [42] ; to our knowledge, no other routes to selectively access such monofluorinated alkenyl thioethers are known. Alternative functionalization also proved possible, such as substitution of both fluorines in 9 by reaction with excess p -methoxyphenol in the presence of NaH, affording the trisubstituted olefin 67 in 42% yield [43] . Fig. 4 Gram-scale synthesis and further transformations. Gram-scale synthesis of product 9 (1). Mono-defluorination of product 9 (2). Double defluorination of product 9 (3) Full size image Mechanistic investigations To gain insight into the reaction mechanism, a CF 3 CHN 2 solution in dichloromethane was prepared according to previous reports (Fig. 5 , Eq. 4) [5] , and then treated with 4-methylbenzenethiol under Method A, which led to 2 and 2′ in 48% and 3% yield respectively as detected by 1 H NMR analysis of the crude reaction mixture. However, if neutral water was used instead of aqueous KOH, only 2′ was obtained (61%). These results suggest that base plays a crucial role in the gem -difluoroalkenylation reaction, in that it may either facilitate reaction of the heteroatomic nucleophile by deprotonation, and/or may promote a β-F elimination of a reaction intermediate. To confirm that the trifluoroethyl sulfide 2′ is indeed a side product rather than an intermediate, conversion of 2′ into 2 under Method A was attempted, but without success (Eq. 5). This may imply that the reaction mechanism involves direct fluoride ion elimination from a carbenoid-derived species, rather than elimination of HF from the trifluoroethyl group. The observation that (2,2,2-trifluoroethoxy)methylbenzene 68 was also not converted to 38 under Method C (Eq. 6) supports this hypothesis. Fig. 5 Mechanistic investigations. Base promotes fluoride elimination (4) Intermediate experience verification (5) and (6) Full size image Proposed mechanism Based on these experimental results, a plausible reaction mechanism is proposed in Fig. 6 in which trifluorodiazoethane is generated in situ from TFHZ-Tfs under the basic reaction conditions, and then reacts with the metal catalyst to form carbenoid intermediate A . The latter is trapped by the substrate (or deprotonated substrate) to form the oxonium ylide B [44] ; Following deprotonation under the basic reaction conditions, the resultant intermediate C undergoes β-fluoride elimination to give the gem -difluoroalkenylation product, regenerating the metal catalyst [34] , [45] . Fig. 6 Proposed mechanism. Mechanistic insights regarding to formation of oxonium ylide and fluoride elimination Full size image Applications of TFHZ-Tfs in Doyle–Kirmse reaction The high efficiency observed in the difluoroalkenylation encouraged us to test the potential of this reagent in other carbenoid transformations. The Doyle–Kirmse reaction of allyl/propargyl thioethers was first studied, where we were delighted to find that reaction of TFHZ-Tfs with allylic thioethers catalyzed by Fe(TTP)Cl delivered the desired CF 3 -substituted homoallyl or alkenyl products in excellent yields (Fig. 7 ) [46] , [47] . This reaction offers a direct and powerful method for the construction of C( sp 3 )–S and C–C bonds by [2,3]-sigmatropic rearrangement of diazo-derived ylids [48] , [49] , and again the use of TFHZ-Tfs proved superior for the generation of trifluorodiazoethane compared to the oxidation of trifluoroethylamine [50] . The scope of this reaction was found to be quite broad, with aryl thioethers containing electron-donating and electron-withdrawing groups at different positions of aryl ring affording CF 3 -substituted homoallyl products ( 69–83 ) in good to excellent yields. Thioethers bearing a disubstituted aryl group also proved suitable, such as a 2,5-dimethylated substituent, which gave product 84 in 84% yield. Naphthyl and heteroaryl allyl thioethers also proceeded efficiently to give the corresponding products 85 and 86 (80% and 75%, respectively). Alkyl allyl thioethers, including benzyl, methyl, and bisallyl substituents, were also well-tolerated to produce the desired products ( 87–89 ) in good yields. Fig. 7 Scope of Doyle–Kirmse reaction. Reaction conditions: thioether (0.3 mmol), TFHZ-Tfs (0.6 mmol), FeTPPCl (3 mol%), NaOH (aq. )/DCM (5:1), 40 °C, 18 h Full size image Scope of Doyle–Kirmse reaction with allyl thioether The effect of substituents (R 1 , R 2 , and R 3 ) on the allyl thioether unit was similarly evaluated, which revealed that the substituent at the 2′-position substituent on the allyl thioether unit (R 1 ) could be varied (methyl, phenyl, or halogen), giving products 90–93 with high efficiency. 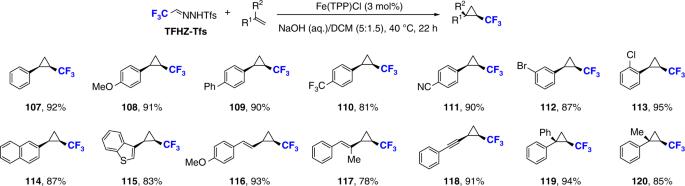Fig. 8 Scope of trifluoromethylcyclopropanation. Reaction conditions: olefin (0.3 mmol), TFHZ-Tfs (0.6 mmol), FeTPPCl (3 mol%), NaOH (aq.)/DCM (5:1.5), 40 °C, 22 h Equally, a range of 1,2-disubstituted allylic thioethers (R 2 = Me/Ph, R 3 = H/Me) were compatible, affording products ( 94–98 ) with high stereoselectivity (up to 10:1 dr , absolute configuration of major isomers was unambiguously confirmed by single crystal X-ray diffraction analysis of its derivatives, details see Supplementary Table 8 ). Most noteworthy among these variations is the rearrangement to generate a quaternary carbon center in homoallylic sulfide 96 . Moreover, a cyclic olefin-substituted thioether afforded the S -to- C transposition product 99 in 77% yield, with high stereoselectivity (7:1 dr ). Scope of Doyle–Kirmse reaction with propargyl thioether We next investigated the scope of the Doyle–Kirmse reaction using propargyl thioethers. Pleasingly, aryl, alkyl, fused aryl, and heteroaryl-functionalized propargyl thioethers all reacted smoothly with TFHZ-Tfs to give the expected allene products in good to excellent yields ( 100 – 103 ). Internal alkynyl thioethers exhibited outstanding reactivity, as demonstrated by reactions of methyl-, phenyl- and TMS-substituted propargyl thioethers, which gave products 104 – 106 in 72–75% yield. Applications of TFHZ-Tfs in cyclopropanation Finally, the application of TFHZ-Tfs as a diazo precursor in cyclopropanation reactions was examined, with the aim of providing an alternative approach to medicinally-relevant trifluoromethylcyclopropanes [2] , [51] , [52] , [53] , [54] , [55] . To our delight, various terminal olefins underwent smooth reaction with TFHZ-Tfs under basic conditions in the presence of Fe(TPP)Cl, giving the desired CF 3 -substituted cyclopropanes in high yields (Fig. 8 ). Good functional group tolerance and excellent stereoselectivity (>20:1) were observed: electron-neutral, -rich, and -poor styrenes all underwent efficient cyclopropanations, affording the corresponding trifluoromethylcyclopropane products 107 – 113 in 81–95% yields. Again, naphthyl and heteroaryl groups were accommodated, providing products 114 and 115 in 87% and 81% yields respectively. Other conjugated dienes and enynes were examined, and also generated the corresponding cyclopropanes ( 116 – 118 ) in excellent yields. Finally, the use of 1,1-disubstituted olefins was equally well-tolerated in spite of increased steric hindrance, delivering trisubstituted products 119 and 120 without diminishing the reaction efficiency or stereoselectivity. Fig. 8 Scope of trifluoromethylcyclopropanation. Reaction conditions: olefin (0.3 mmol), TFHZ-Tfs (0.6 mmol), FeTPPCl (3 mol%), NaOH (aq. )/DCM (5:1.5), 40 °C, 22 h Full size image In summary, we report the development of trifluoroacetaldehyde N-tfsylhydrazone (TFHZ-Tfs)—a bench-stable crystalline reagent that represents a versatile trifluorodiazoethane surrogate, which can generate CF 3 CHN 2 under basic conditions in a controlled manner that avoids excessive buildup of the hazardous diazo compound. A number of applications of TFHZ-Tfs are described, including the discovery of gem -difluoroalkenylation of X–H bonds (X = S, N, O, Se), Doyle–Kirmse rearrangements, and trifluoromethylcyclopropanation reactions, with superior performance over other sources of CF 3 CHN 2 . Considering the procedural advantages of this trifluorodiazoethane surrogate, and the importance of generally applicable fluorination methodologies, these findings create many opportunities for the wider exploration of the chemistry of trifluorodiazoethane. General procedure for the synthesis of gem -difluorovinyl thioether A screw capped reaction vial was charged with TFHZ-Tfs (0.6 mmol), toluenethiol (0.3 mmol), Fe[P2] (0.003 mmol) and SDBS (sodium dodecylbenzenesulphonate) (0.09 mmol) under air, followed by addition of DCM (1.0 mL) and KOH aq. (5.0 mL, 20 wt%) (Fig. 5 , Method A) . The resulting mixture was stirred at 40 °C for 18 h. Then 10 mL water was added to the mixture, which was extracted with DCM (3 × 10 mL). The organic layer was combined and dried with anhydrous MgSO 4 , then filtered through a short silica gel eluting with DCM. The filtrate was evaporated under reduced pressure to leave a crude mixture, which was separated by flash column chromatography to afford the pure product. General procedure for the synthesis of gem -difluorovinyl amine A screw capped reaction vial was charged with TFHZ-Tfs (0.6 mmol), amine (0.3 mmol), Cu(OTf) 2 (0.06 mmol) and LiO t Bu (1.2 mmol), then evacuated and filled with argon for three times, followed by addition of DCE (3.0 mL) and toluene (1.0 mL) via syringe (Fig. 5 , Method B). The resulting mixture was stirred at 40 °C for 24 h. The reaction crude was filtered through a short silica gel eluting with DCM. The filtrate was evaporated under reduced pressure to leave a crude mixture, which was separated by flash column chromatography to afford the pure product. General procedure for the synthesis of gem -difluorovinyl ether A screw capped reaction vial was charged with TFHZ-Tfs (1.0 mmol), and NaH (60 wt%, 2 mmol) and was evacuated and filled with argon for three times, followed by addition of dry DCE (8.0 mL) via syringe. The resulting mixture was stirred at room temperature for 1 h (Fig. 5 , Method C). Then, alcohol (0.5 mmol) and CuBr (0.15 mmol) were added and the system was stirred at 40 °C for 24 h. The reaction crude was filtered through a short silica gel eluting with DCM. The filtrate was evaporated under reduced pressure to leave a crude mixture, which was purified by column chromatography on silica gel. General procedures for Doyle–Kirmse reaction A screw capped reaction vial was charged with TFHZ-Tfs (0.6 mmol), FeTPPCl (0.009 mmol), then evacuated and filled with argon for three times, then DCM (1 mL) which dissolved with allyl or propargyl sulfide (0.3 mmol) and NaOH aq. (5 mL, 20 wt%) was successively added by syringe (Fig. 7 ). The reaction was stirred at 40 °C for 18 h. Then 10 mL water was added to the mixture and layers partitioned. The aqueous layer was extracted with DCM (3 × 10 mL) and the organic layer was combined and dried with anhydrous MgSO 4 , then filtered through a short silica gel eluting with DCM. The filtrate was evaporated under reduced pressure to leave a crude mixture, which was purified through silica gel flash column chromatography eluting with n -hexane to give the final product. General procedures for cyclopropanation reaction A screw capped reaction vial was charged with TFHZ-Tfs (0.6 mmol), FeTPPCl (0.009 mmol), then evacuated and filled with argon for three times, then DCM (1.5 mL) which dissolved with styrene (0.3 mmol) and NaOH aq. (5 mL, 20 wt%) was successively added by syringe (Fig. 8 ). The reaction was stirred at 40 °C for 22 h. Then 10 mL water was added to the mixture and layers partitioned. The aqueous layer was extracted with DCM (3 × 10 mL) and the organic layer was combined and dried with anhydrous MgSO 4 , then filtered through a short silica gel eluting with DCM. The filtrate was evaporated under reduced pressure to leave a crude mixture, which was purified through silica gel flash column chromatography eluting with n -hexane to give the final cyclopropane product.